Sign-reversal of the in-plane resistivity anisotropy in hole-doped iron pnictides Unconventional superconductivity usually originates from several strongly coupled degrees of freedom, such as magnetic, charge and elastic. A highly anisotropic electronic phase, not driven by lattice degrees of freedom, has been proposed in some of these superconductors, from cuprates to iron-based compounds. In the iron pnictide BaFe 2 As 2 , this nematic phase arises in the paramagnetic phase and is present for wide doping and temperature ranges. Here we probe the in-plane electronic anisotropy of electron- and hole-doped BaFe 2 As 2 compounds. Unlike other materials, the resistivity anisotropy behaves very differently for electron- and hole-type dopants and even changes sign on the hole-doped side. This behaviour is explained by Fermi surface reconstruction in the magnetic phase and spin-fluctuation scattering in the paramagnetic phase. This unique transport anisotropy unveils the primary role played by magnetic scattering, demonstrating the close connection between magnetism, nematicity and unconventional superconductivity. Two decades of intense research have shown that unconventional superconductors, including those with particularly high critical temperatures, T c , often neighbour antiferromagnetic phases. It is believed that while long-range magnetic order is detrimental to superconductivity, magnetic fluctuations can be instrumental in assisting to form the Cooper pairs. In iron-based superconductors, proximity to stripe-type magnetic order is particularly prominent, and these two phases even coexist in some compounds. Interestingly, the transition to the long-range magnetically ordered phase is preceded or accompanied by a structural transition (see Paglione and Greene [1] , and Johnston [2] for review). In the family of A Fe 2 As 2 ( A =Ca, Sr, Ba, Eu) compounds, the stripe magnetic order below T N breaks tetragonal symmetry [3] , with in-plane ordering vectors (π,0) or (0,π). The structural transition at T S ≥ T N preempts the magnetic one and reduces the tetragonal symmetry of the lattice to orthorhombic. It has been suggested by several experiments [4] , [5] , [6] , [7] and theories [8] , [9] , [10] , [11] , [12] that the tetragonal symmetry breaking is caused by magnetic, that is, electronic, rather than elastic degrees of freedom, giving rise to the so-called electronic nematic phase [13] . In a broader context, electronic nematicity has been experimentally observed in many systems such as semiconductor heterostructures [14] , ruthenates [15] , cuprate [16] and iron pnictide [4] superconductors. In BaFe 2 As 2 , doping with either electrons (by Co-substitution of Fe, Ba(Fe 1− x Co x ) 2 As 2 ) or holes (by K-substitution of Ba, (Ba 1− x K x )Fe 2 As 2 ) suppresses both magnetic and nematic orders, revealing superconductivity with a maximum T c close to the edges of the magnetic/nematic dome ( Fig. 1 ). 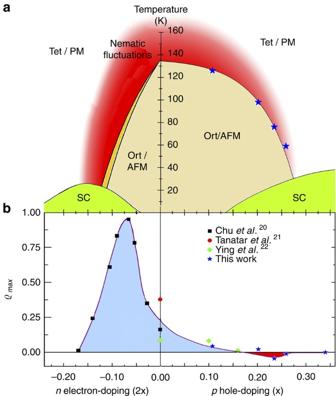Figure 1: Doping phase diagram and resistivity anistropy. (a) Phase diagram of the electron- and hole-doped Ba122 system focusing on the under-doped regime with the superconducting (SC) region shown in green. The yellow region denotes the orthorhombic/antiferromagnetic (Ort/AFM) phase below the transition from tetragonal/paramagnetic (Tet/PM) phase atTS. Nematic fluctuations (red region) persist far aboveTSand affect the in-plane resistivity anisotropy in strained samples. (b) The maximum in-plane anisotropyρmaxas a function of doping. Note the significant asymmetry ofρmax(x) and its sign-change in the hole-doped regime. Figure 1: Doping phase diagram and resistivity anistropy. ( a ) Phase diagram of the electron- and hole-doped Ba122 system focusing on the under-doped regime with the superconducting (SC) region shown in green. The yellow region denotes the orthorhombic/antiferromagnetic (Ort/AFM) phase below the transition from tetragonal/paramagnetic (Tet/PM) phase at T S . Nematic fluctuations (red region) persist far above T S and affect the in-plane resistivity anisotropy in strained samples. ( b ) The maximum in-plane anisotropy ρ max as a function of doping. Note the significant asymmetry of ρ max ( x ) and its sign-change in the hole-doped regime. Full size image Below T S , the sample splits into structural twin domains with different directions of the orthorhombic a 0 and b 0 axes (a 0 >b 0 ) ( [17] ). Applying a small uniaxial strain not only stabilizes one particular domain below T S , but also extends the nematic phase to temperatures well above T S , due to the coupling between the strain field and nematic fluctuations (red area in Fig. 1 ) ( [7] , [18] , [19] ). In these strained samples, the nematic state anisotropy reveals itself not only in the small orthorhombic distortion a 0 −b 0 <<a 0 +b 0 , but, more so, in a pronounced anisotropy of the in-plane electrical resistivity ρ ≡ ρ b / ρ a −1 ( [20] , [21] , [22] ). Regardless of the microscopic nature of the nematic order parameter, φ , symmetry imposes that close to the nematic transition temperature, ρ = κφ , where κ is a coupling parameter. Indeed, this relation was verified experimentally in the parent compound of BaFe 2 As 2 ( [18] ). Not surprisingly, in the only system where the electronic anisotropy was systematically studied across the nematic dome, the ruthenate Sr 3 Ru 2 O 7 ( [15] ), ρ was found to retain the same sign across the phase diagram. In the quantum Hall system of Cooper et al . [14] , on the other hand, the resistivity anisotropy was found to change sign for a particular direction of the external symmetry-breaking field, a behaviour that remains without clear microscopic interpretation. In the BaFe 2 As 2 family, most of the studies on its nematicity have focused on the electron-doped compounds, finding ρ >0 in both magnetic and nematic phases [20] , [21] , [23] . More recently, experiments in under-doped (Ba 1− x K x )Fe 2 As 2 found a rather small, but still positive, value of ρ [22] . Here we report that for larger K-doping levels, not explored in the previous studies, the anisotropy ρ changes sign both near T S (nematic phase) and at very low temperatures (magnetically ordered phase). As the sign of φ is fixed by the small applied uniaxial strain, the coupling parameter κ must change sign across the magnetic/nematic dome. We interpret this sign-change as a result of asymmetric changes in the magnetic scattering and in the magnetically reconstructed band structure for electron- and hole-doping. This unique complexity of the nematic dome observed in the iron pnictides, suggests that spin-scattering dominates transport in the normal state, establishing a possible connection to a magnetically mediated mechanism of superconductivity. 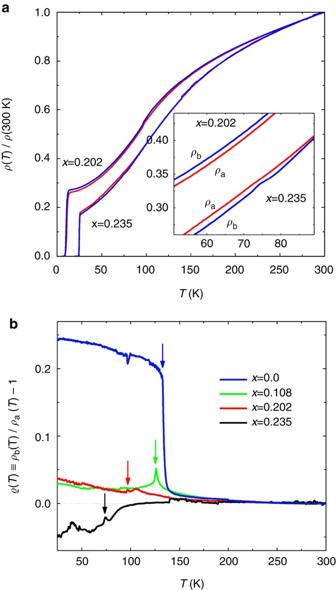Figure 2: Sign-change of the resistivity anisotropy. (a) Normalized temperature-dependent resistivity,ρ(T)/ρ(300K), for the (Ba1−xKx)Fe2As2samples withx=0.202 andx=0.235. The red lines show the resistivity along thea0-axis (ρa) while the blue lines showρb. The inset zooms at the structural transition, where a clear reversal of the anisotropy fromρb>ρaforx=0.202 toρb<ρaforx=0.235 occurs. (b) Temperature dependence ofρfor different K-doping levels. Arrows showTNdetermined from dρ(T)/dTon unstrained samples. Sign-change of resistivity anisotropy Figure 2 presents our main experimental finding, the sign-reversal of the in-plane resistivity anisotropy. For (Ba 1− x K x )Fe 2 As 2 samples with x ≤0.202, the resistivity is larger along the shorter orthorhombic axis, ρ a < ρ b , whereas for samples with x ≥0.235, the longer axis has higher resistivity, ρ a > ρ b . This is clearly seen in the inset zooming in on the structural transition region. It is also apparent that, because of the applied uniaxial strain, the in-plane anisotropy starts to appear well above the structural transition T S of the unstrained sample. Figure 2: Sign-change of the resistivity anisotropy. ( a ) Normalized temperature-dependent resistivity, ρ ( T )/ ρ (300 K ), for the (Ba 1− x K x )Fe 2 As 2 samples with x =0.202 and x =0.235. The red lines show the resistivity along the a 0 -axis ( ρ a ) while the blue lines show ρ b . The inset zooms at the structural transition, where a clear reversal of the anisotropy from ρ b > ρ a for x =0.202 to ρ b < ρ a for x =0.235 occurs. ( b ) Temperature dependence of ρ for different K-doping levels. Arrows show T N determined from d ρ ( T )/d T on unstrained samples. Full size image In Fig. 2b , we plot the temperature-dependent anisotropy ratio, ρ , for several compositions. We use two characteristic features of the ρ ( T ) curves to further analyse the data. First, we plot in Fig. 1b the maximum in-plane anisotropy ρ max for different x . In Fig. 3a we plot ρ ( T ≈ T N ), that is, at temperatures immediately below the magnetic transition, which coincides with the structural transition temperature of the unstrainned (Ba 1− x K x )Fe 2 As 2 samples. 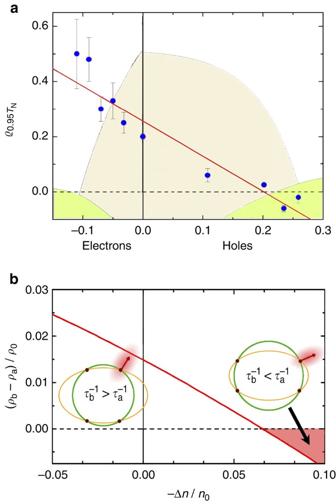Figure 3: Anisotropic scattering from spin fluctuations. (a) Doping dependence of the in-plane resistivity anisotropy at 0.95TNin both electron- and hole-doped BaFe2As2. The red line is a guide to the eye. The nematic/magnetic and superconducting domes are shown in the background for reference only, without a temperature scale. The error bars represent the values of the resistivity anisotropy ratio atTNand reflect the uncertainty in the determination ofTNfrom the maximum of the dρ(T)/dTcurves. (b) Theoretical calculation of the maximum in-plane resistivity anisotropy in the paramagnetic phase normalized by the residual resistivity,ρ0, as a function of the change in the electron occupation number, Δn/n0, wheren0=(kFa)2/(π). The insets schematically show the differences in the scattering rates corresponding to different Fermi velocities at the hot-spots for electron- and hole-doped systems. When the hot-spot Fermi velocity has a larger component along theb(a) direction, the magnetic scattering rate is larger along theb(a) direction. The hot-spots are obtained by displacing the electron pocket (yellow ellipse) by (π,0), making it overlap with the hole pocket (green circle). The shaded red area denotes the predicted sign-reversal of the anisotropy. Figure 3: Anisotropic scattering from spin fluctuations. ( a ) Doping dependence of the in-plane resistivity anisotropy at 0.95 T N in both electron- and hole-doped BaFe 2 As 2 . The red line is a guide to the eye. The nematic/magnetic and superconducting domes are shown in the background for reference only, without a temperature scale. The error bars represent the values of the resistivity anisotropy ratio at T N and reflect the uncertainty in the determination of T N from the maximum of the d ρ ( T )/d T curves. ( b ) Theoretical calculation of the maximum in-plane resistivity anisotropy in the paramagnetic phase normalized by the residual resistivity, ρ 0 , as a function of the change in the electron occupation number, Δ n / n 0 , where n 0 =( k F a ) 2 /( π ). The insets schematically show the differences in the scattering rates corresponding to different Fermi velocities at the hot-spots for electron- and hole-doped systems. When the hot-spot Fermi velocity has a larger component along the b ( a ) direction, the magnetic scattering rate is larger along the b ( a ) direction. The hot-spots are obtained by displacing the electron pocket (yellow ellipse) by (π,0), making it overlap with the hole pocket (green circle). The shaded red area denotes the predicted sign-reversal of the anisotropy. Full size image This sign-change happens at all temperatures, even near T N , as shown in Fig. 2b and in Fig. 3a . Furthermore, as it can be seen in Fig. 2b , the magnitude of the temperature-dependent anisotropy ratio, ρ ( T ), is maximal close to T N in the parent and slightly hole-doped compositions, but increases monotonically on cooling for higher hole doping levels. This signals that the low-temperature anisotropic reconstruction of the band structure due to long-range magnetic order has a progressively more important role near the hole-doped edge of the nematic/magnetic dome. Electron versus hole doping An interesting general picture emerges from the analysis of the experimental observations of this and previous studies [20] , [21] , [22] . On the one hand, for all electron-doped Ba(Fe 1− x Co x ) 2 As 2 and parent compositions, the resistivity anisotropy is positive, ρ ( x )>0. The maximum anisotropy, ρ max ( x ), shown in Fig. 1b , is peaked at some intermediate electron doping, vanishing near the edge of the magnetic/nematic dome, due to the vanishing orthorhombic distortion. On the other hand, on the hole-doped side, ρ max ( x ) remains positive up to moderate hole doping, but decreases by more than one order of magnitude, from ρ max ( x =0)≈+0.3 to ρ max ( x =0.202)≈+0.02. Even more surprisingly, ρ max ( x ) changes sign and exhibits a minimum at a higher hole doping concentration, ρ max ( x =0.235)≈−0.034, before it eventually approaches zero close to the edge of the magnetic/nematic dome, near x =0.3. Naively, the fact that ρ b > ρ a across most of the phase diagram seems surprising, because the ferromagnetic direction appears to be less conducting than the antiferromagnetic one. From the orbital ordering point of view [11] , [24] , [25] one expects the opposite effect. However, a closer look at the Fermi surface reconstruction [21] , [23] and the magnetic scattering mechanisms [26] , [27] suggests that the anisotropy sign is decided by quantitative factors that depend on the electronic structure, going beyond general order parameter arguments. Moreover, the different contributions to the transport anisotropy do not necessarily compete with each other. To sort them out, we focus first on the nematic paramagnetic phase, in which scattering by magnetic fluctuations dominates and the band structure is not yet reconstructed by the magnetic order. The experimental doping evolution of ρ ( T ≈ T N ), shown in Fig. 3a displays a rather monotonic behaviour, changing sign for sufficient hole-doping levels and vanishing at the edges of the nematic dome. Such a sign-change was previously predicted by the theoretical model of Fernandes et al . [26] for the anisotropic magnetic scattering in the nematic phase. The minimal model of Fernandes et al . [26] , shown in the Supplementary Note 1 to be consistent with first-principles calculations, consists of a circular hole pocket at the center of the square-lattice Brillouin zone and two elliptical electron pockets centred at momenta (π,0) and (0,π), which coincide with the magnetic-stripe ordering vectors (see Supplementary Figs S1 and S2 ). In the nematic phase, the amplitude of the fluctuations around these two ordering vectors becomes unequal [12] , breaking the tetragonal symmetry of the system and inducing anisotropic scattering. In the experiment, the applied strain selects the (π,0) fluctuations. The work by Fernandes et al . [26] showed that in the presence of impurities and in the low-temperature limit—but still in the paramagnetic phase—the scattering rates along a and b (and consequently the sign of the resistivity anisotropy) is controlled by the Fermi velocities of the hot-spots connecting the hole and electron pockets, see Fig. 3 . Roughly in electron-doped compounds, the hot-spots Fermi velocity has a larger component along the b direction, giving rise to a larger scattering rate for electrons travelling along this direction, implying ρ b > ρ a . As the system is doped with holes, the hole pocket expands while the electron pocket shrinks, changing the position and the Fermi velocity of the hot-spots, which eventually acquires a larger component along the a direction, implying ρ a > ρ b . Although Fermi velocity measurements in detwinned hole-doped samples are not available, angle-resolved photoemission spectroscopy data in optimally Co-doped [28] and K-doped [29] twinned samples support such a change in the direction of the Fermi velocity at the hot-spots. The existence of hot-spots in optimally K-doped samples is also strongly supported by inelastic neutron scattering data, displaying overdamped-like behaviour in the normal state that disappears in the superconducting phase, where hot-spot electron states are gapped [30] . To go beyond the low-temperature paramagnetic limit and make closer connection to the experiment, we used the same model of Fernandes et al . [26] and numerically obtained the maximum resistivity anisotropy in the paramagnetic phase as function of doping. The results, shown in Fig. 3b , agree qualitatively with the experimental data, capturing both the electron-hole asymmetry of ρ ( T ≈ T N ) and its sign-change in the hole-doped regime. This suggests that magnetic scattering has a central role in the paramagnetic phase. Our data in Fig. 2 also show that the sign-change in the resistivity anisotropy persists down to T =0, deep inside the magnetic state, where magnetic fluctuations are weaker. In this regime, transport should be governed by anisotropic reconstruction of the band structure. By employing first-principles calculations, we obtained the Fermi surface in the magnetically ordered state and evaluated ρ in the relaxation-time approximation (see Supplementary Note 2 ). Our calculations show that, in the parent compound, the reconstructed Fermi surface contains not only quasi-isotropic hole and electron pockets, but also Dirac cones whose crossing points are located slightly below the Fermi level ( Supplementary Fig. S3 ). These features are in good agreement with quantum oscillation measurements [23] . Owing to the large value of their Fermi velocities, these Dirac cones dominate the transport in the magnetic state, giving rise to an anisotropy in the resistivity that is in agreement with the experimental observations for x =0. When holes are added to the system, the chemical potential shifts down, eventually crossing the Dirac points. Using the values extracted by angle-resolved photoemission spectroscopy [31] , [32] and quantum oscillation measurements [23] , we estimate this Dirac-point crossing to happen between 0.03 and 0.1 holes/Fe. For this doping concentration, the contribution to ρ coming from the Dirac pockets is vanishingly small, making the contribution from the remaining pockets dominant (see Supplementary Figs S4 and S5 ). The latter depends on details that are beyond the accuracy of first-principles calculations, and can either yield a small positive or negative ρ . Yet, our first-principles approach correctly captures the tendency of a vanishing ρ inside the magnetically ordered phase in the hole-doped samples. In conclusion, we observe the reversal of the in-plane resistivity anisotropy between electron- and hole-doped BaFe 2 As 2 compounds. We attribute such behaviour to the spin-fluctuation scattering in the nematic phase and to the Dirac-cones contribution in the magnetically ordered phase. Both mechanisms complementarily predict a resistivity anisotropy that is larger in the electron-doped side and continuously smaller in the hole-doped side. We notice that other contributions not considered here, such as anisotropic impurity potential or anisotropic defects, can also affect the transport anisotropy in the iron pnictides. Our analysis offers an explanation for the change in the sign of the resistivity anisotropy in terms of the band structure of the pnictides, without invoking a change from itinerant to local moment physics, as suggested recently by Jiang et al . [33] Interestingly, the changes in the band structure from electron to hole-doped compounds [34] , [35] also cause a reversal of the anisotropy in the magnetic correlation length [30] , which, however, has little impact on the sign-changing of the resistivity anisotropy within our model [26] . Besides shedding light on the singular character of the nematic phase in the iron pnictides, our observation serves as a unique fingerprint for the predominance of electronic scattering due to spin fluctuations, rather than phonons, in the normal state of these superconductors. Therefore, our study provides strong support to the concept that anomalous magnetic scattering in the proximity of a putative quantum critical point is intimately connected to magnetically mediated unconventional superconductivity [36] , [37] . Crystal growth and characterization Single crystals of (Ba 1− x K x )Fe 2 As 2 with a size up to 7 × 7 × 1 mm 3 were grown from FeAs flux as described in Luo et al . [38] Potassium content in the samples was determined using electron probe microanalysis with wavelength dispersive spectroscopy, see Tanatar et al . [39] for details. Samples, had typical dimensions of 0.5 mm wide, 2–3 mm long and 0.05 mm thick, and were cut from cleaved slabs along the tetragonal [110] direction (which becomes either the orthorhombic a 0 or b 0 axis below T SM ). Optical imaging was performed on the samples while mounted on a cold finger in a continuous flow liquid helium cryostat (allowing for precise temperature control in 5 K to 300 K range) using a Leica DMLM microscope. Polarized light microscopy was used for visualization of the structural domains [17] and the sample selection was based on the clarity of domains in the image. In Fig. 4 , we show polarized light images of the area between potential contacts in (Ba 1− x K x )Fe 2 As 2 crystals used in this study, with x =0.108 (non-superconducting), x =0.202 ( T c =10 K), x =0.235 ( T c =26 K) and x =0.259 ( T c =28 K). Images were taken on cooling at a temperature slightly above T s and at base temperature. The highest contrast is observed when the sample is aligned with the [100] tetragonal direction at a 45° to the polarization direction of incident light (parallel and perpendicular to the orthorhombic a 0 in different domains). The contrast of domain images depends on the quality of the surface and the homogeneity of the samples. Domains are observed for samples with x ≈0.26, and are no longer observed for samples with a higher doping level, x =0.34, which also do not show any features associated with a structural transition in ρ ( T ). 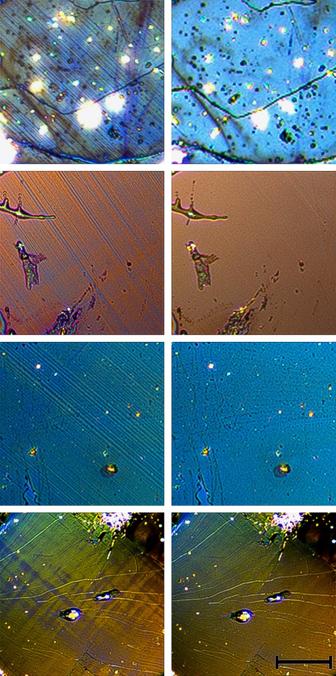Figure 4: Visualization of structural domains. Polarized light microscopy of (Ba1−xKx)Fe2As2samples with doping levelsx=0.108, 0.202, 0.235, 0.259, from top to bottom. Images were taken at temperatures just above the tetragonal-to-orthorhombic structural transition (T>TS, right) and 5 K (T<TS, left), the latter showing formation of structural domains due to four different orientations ofa0andb0axes. The difference in colour of the domains is due to spectral dependence of bireflectance, depending on angle between the a0direction and the polarization plane of incident white light. As bireflectance is proportional to the orthorhombic distortion, the contrast naturally vanishes in the tetragonal phase (right panels). Scale bar, 100 μm. Figure 4: Visualization of structural domains. Polarized light microscopy of (Ba 1− x K x )Fe 2 As 2 samples with doping levels x =0.108, 0.202, 0.235, 0.259, from top to bottom. Images were taken at temperatures just above the tetragonal-to-orthorhombic structural transition ( T > T S , right) and 5 K ( T < T S , left), the latter showing formation of structural domains due to four different orientations of a 0 and b 0 axes. The difference in colour of the domains is due to spectral dependence of bireflectance, depending on angle between the a 0 direction and the polarization plane of incident white light. As bireflectance is proportional to the orthorhombic distortion, the contrast naturally vanishes in the tetragonal phase (right panels). Scale bar, 100 μm. Full size image Resistivity measurements and mechanical detwinning Selected samples were mounted for four-probe electrical resistivity measurements, with contacts made by soldering 50 μm Ag wires using low-resistance Sn soldered contacts [40] . Initial resistivity measurements on each sample were carried out using a flexible wire arrangement with no strain applied to the sample (free standing state). The results are plotted in Fig. 5 . As this measurement is performed in the twinned state of the sample and contains contributions from both components of the in-plane resistivity in the orthorhombic phase, we call it ρ t . Samples were then mounted on a brass horseshoe straining device, and strain was applied through the voltage contact wires by deformation of the horseshoe, see Tanatar et al . [21] and Blomberg et al . [41] for the details of the procedure. Strain in this configuration is applied along the tetragonal [110] axis, which selects the orthorhombic a 0 -axis as a preferable direction upon cooling below T S . Very soft current leads apply no strain. The strain was incrementally increased, and for each increment, temperature-dependent resistivity measurements were made and the domain structure was imaged to determine the completeness of detwinning. Our previous studies [18] , [21] using x-ray scattering have shown that when crystals are strained to the point at which no domains are visible in polarized microscopy, about 90% of the whole bulk of the sample represents the domain whose orthorhombic a 0 -axis is oriented along the direction of the strain and, therefore, parallel to the current. Therefore, in the detwinned state we are predominantly measuring the a 0 -axis resistivity, ρ a , while in the unstrained state of the sample roughly equal contributions of both resistivity components are measured. Therefore, we may calculate the b 0 axis resistivity, ρ b ( T )=2 ρ t ( T )− ρ a ( T ). 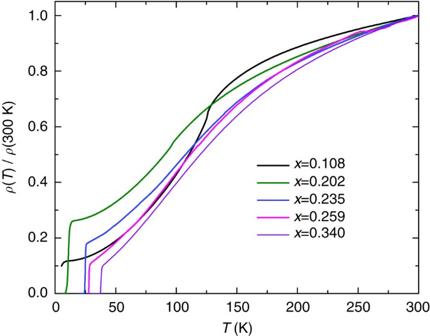Figure 5: Temperature-dependent resistivity. Temperature-dependent resistivity along the orthorhombica0-axis,ρafor samples of (Ba1−xKx)Fe2As2with four different potassium doping levels in the strain-free, twinned state. The curves are shown using normalized plots,ρ(T)/ρ(300 K). Figure 5: Temperature-dependent resistivity. Temperature-dependent resistivity along the orthorhombic a 0 -axis, ρ a for samples of (Ba 1− x K x )Fe 2 As 2 with four different potassium doping levels in the strain-free, twinned state. The curves are shown using normalized plots, ρ ( T )/ ρ (300 K). Full size image How to cite this article: Blomberg, E. C. et al . Sign-reversal of the in-plane resistivity anisotropy in hole-doped iron pnictides. Nat. Commun . 4:1914 doi: 10.1038/ncomms2933 (2013).